Multi-body coalescence in Pickering emulsions Particle-stabilized Pickering emulsions have shown unusual behaviours such as the formation of non-spherical droplets and the sudden halt of coalescence between individual droplets. Here we report another unusual behaviour of Pickering emulsions—the simultaneous coalescence of multiple droplets in a single event. Using latex particles, silica particles and carbon nanotubes as model stabilizers, we show that multi-body coalescence can occur in both water-in-oil and oil-in-water emulsions. The number of droplets involved in the n th coalscence event equals four times the corresponding number of the tetrahedral sequence in close packing. Furthermore, coalescence is promoted by repulsive latex and silica particles but inhibited by attractive carbon nanotubes. The revelation of multi-body coalescence is expected to help better understand Pickering emulsions in natural systems and improve their designs in engineering applications. Pickering emulsions are made of particle-stabilized droplets suspended in an immiscible continuous liquid phase [1] , [2] . They are important soft matter systems that form naturally in crude oils [3] and food products [4] and have been engineered for drug delivery [5] , water purification [6] and material processing [7] , [8] , [9] , [10] . Compared with ordinary emulsions, Pickering emulsions are distinctively stable because the removal of interfacial particles requires a large amount of energy [11] . When individual Pickering droplets are forced to coalesce, the extraordinary stability brought about by interfacial particles can lead to the formation of non-spherical droplets [12] , [13] , [14] and the arrest of droplet coalescence [15] , [16] . Little is known, however, about the coalescence of a collection of hundreds and thousands of Pickering droplets as in real emulsions. This is particularly important when particle stabilizers are used to produce near-monodispersed droplets [17] , during which the distribution of droplet size can be significantly broadened by coalescence under gravity, floatation and shear [18] , [19] . Here we report for the first time that the presence of stabilizers at the oil–water interface can lead to multi-body coalescence in an ensemble of Pickering droplets—a phenomenon that has not been reported for either Pickering or ordinary emulsions. More interestingly, the number of droplets involved in coalescence equals four times the corresponding number of the tetrahedral sequence, indicating the inclusion of all closely packed nearest neighbours in a single coalescene event. As a result, a magic size distribition is produced with distinctive maxima related to each other through the cubic root of four times the tetrahedral numbers. Futhermore, interactions between stabilizers are found to affect the probability of coalescence by varying interfacial tension. Using model stabilizers including latex particles, silica particles and carbon nanotubes (CNTs), we show that coalescence is promoted by interparticle repulsion but inhibited by interparticle attraction. Selection of emulsion systems To investigate coalescence of Pickering droplets in an ensemble, we select three representative emulsion systems, including latex particle-stabilized water droplets in dodecane, silica particle-stabilized 1,2-dichlorobenzene (DCB) droplets in water and CNT-stabilized water droplets in dodecane. Comparisons between the first two systems will show that multi-body coalescence occurs in both water-in-oil and oil-in-water emulsions. Subsequent comparisons with the CNT system will reveal differences between stabilizers lacking and having attractive interactions. Our results are organized in four sections as follows, including emulsion preparation and droplet size analysis, evolution of droplet size through multi-body coalescence, polydispersity and size evolution and coalescence probability and interparticle force. Emulsion preparation and droplet size analysis The three stabilizers and typical Pickering emulsions made from them are shown in Fig. 1 . Latex and silica particles ( Fig. 1a,b ) are spheres with diameters of 0.8 μm and 1 μm, respectively. CNTs decorated with surface tension-tuning magnetite (Fe 3 O 4 ) nanoparticles ( Fig. 1c ) are several micrometers long and have a diameter of ca. 15 nm (ref. 6 ). Pickering emulsions stabilized by latex particles, silica particles and CNTs are prepared following a conventional protocol [20] , involving two consecutive steps. First, water, oil and stabilizers are mixed and then shaken vigorously by hand for 10 min ( Fig. 1d–f ), forming Pickering emulsions containing stabilizer-wrapped droplets [21] . Then, emulsions are left standing undisturbed on top of a bench for 10 min, allowing droplets to precipitate ( Fig. 1g–i ), forming a closely packed ensemble ( Fig. 1j–l ) to induce coalescence. Pickering droplets prepared following this protocol have low uniformity indices between 0.2 and 0.4 ( Supplementary Fig. 1 ) [22] , [23] , [24] , suggesting that the emulsions have only experienced limited coalescence [21] . 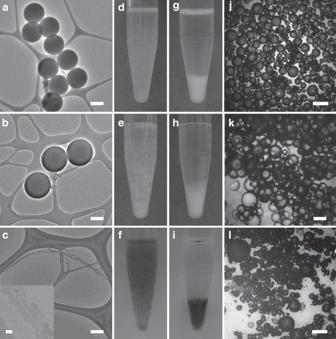Figure 1: Pickering emulsions made of three types of stabilizers. Results obtained with different analytical techniques are organized in columns: (a–c) transmission electron micrographs of stabilizers, (d–f) digital photographs of emulsions during mixing, (g–i) photographs taken at the end of standing and (j–l) optical micrographs of emulsions after standing. Results obtained with different stabilizers are organized in rows: (a,d,g,j) latex particle-stabilized water droplets in dodecane, (b,e,h,k) silica particle-stabilized 1,2-dichlorobenzene (DCB) droplets in water and (c,f,i,l) carbon nanotube-stabilized water droplets in dodecane. Mass ratio between droplets and the continuous phase: (d,g,j), 0.0667; (e,h,k), 0.0650; (f,i,l), 0.0667. Stabilizer-to-droplet mass ratio: (d,g,j), 0.02; (e,h,k), 0.03; (f,i,l), 0.02. Scale bars:a–c, 500 nm; inset inc, 5 nm andj–l, 250 μm. Figure 1: Pickering emulsions made of three types of stabilizers. Results obtained with different analytical techniques are organized in columns: ( a – c ) transmission electron micrographs of stabilizers, ( d – f ) digital photographs of emulsions during mixing, ( g – i ) photographs taken at the end of standing and ( j – l ) optical micrographs of emulsions after standing. Results obtained with different stabilizers are organized in rows: ( a , d , g , j ) latex particle-stabilized water droplets in dodecane, ( b , e , h , k ) silica particle-stabilized 1,2-dichlorobenzene (DCB) droplets in water and ( c , f , i , l ) carbon nanotube-stabilized water droplets in dodecane. Mass ratio between droplets and the continuous phase: ( d , g , j ), 0.0667; ( e , h , k ), 0.0650; ( f , i , l ), 0.0667. Stabilizer-to-droplet mass ratio: ( d , g , j ), 0.02; ( e , h , k ), 0.03; ( f , i , l ), 0.02. Scale bars: a – c , 500 nm; inset in c , 5 nm and j – l , 250 μm. Full size image After coalescence is complete, diameters of at least 500 droplets are measured using an optical microscope. Histograms, as shown in Fig. 2a–c , are constructed to facilitate detailed analyses of droplet size distribution. For all three types of emulsions, the diameter histogram can be readily deconvoluted into a series of Gaussian functions, indicating that each emulsion consists of several normally distributed populations of droplets. Of note, deconvolution is only possible when histograms are generated using at least 500 measurements. Similar histograms reported in the literature are usually made with significantly less measurements, often in the order of 50–100 (ref. 21 ). Under such conditions, the combination of multiple normal distributions degenerates to a single log-normal distribution [25] . 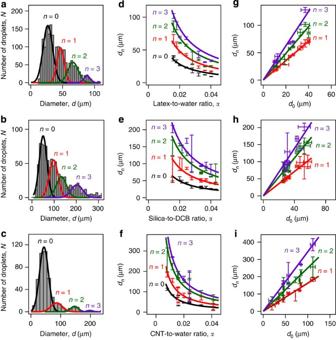Figure 2: Size distributions of three types of Pickering droplets. Results of different analyses are organized in columns: (a–c) diameter histograms showing distinctive maxima:dn's (n=0, 1, 2, 3), (d–f) inverse correlations ofdn's with stabilizer-to-droplet mass ratioαand (g–i) linear correlations ofdn's (n>0) withd0. Results for different stabilizers are organized in rows: (a,d,g) latex particle-stabilized water droplets in dodecane, (b,e,h) silica particle-stabilized 1,2-dichlorobenzene (DCB) droplets in water and (c,f,i) carbon nanotube-stabilized water droplets in dodecane. Curves ind–fare least-square regressions to equation (1). Lines ing–iare regressions to equation (2). Mass ratio between droplets and the continuous phase: (a,d,g), 0.0667; (b,e,h), 0.0650; (c,f,i), 0.0667. Stabilizer-to-droplet mass ratio:a, 0.02;b, 0.03 andc, 0.02. Error bars represent s.e. Figure 2: Size distributions of three types of Pickering droplets. Results of different analyses are organized in columns: ( a – c ) diameter histograms showing distinctive maxima: d n 's ( n =0, 1, 2, 3), ( d – f ) inverse correlations of d n 's with stabilizer-to-droplet mass ratio α and ( g – i ) linear correlations of d n 's ( n >0) with d 0 . Results for different stabilizers are organized in rows: ( a , d , g ) latex particle-stabilized water droplets in dodecane, ( b , e , h ) silica particle-stabilized 1,2-dichlorobenzene (DCB) droplets in water and ( c , f , i ) carbon nanotube-stabilized water droplets in dodecane. Curves in d – f are least-square regressions to equation (1). Lines in g – i are regressions to equation (2). Mass ratio between droplets and the continuous phase: ( a , d , g ), 0.0667; ( b , e , h ), 0.0650; ( c , f , i ), 0.0667. Stabilizer-to-droplet mass ratio: a , 0.02; b , 0.03 and c , 0.02. Error bars represent s.e. Full size image The mean of each deconvoluted normal distribution, d n ( n =0, 1, 2, 3), represents the mean diameter of the corresponding droplet population. We find that d n decreases with increasing stabilizer-to-droplet mass ratio α , as shown in Fig. 2d–f . The inverse dependence of d n on α can be readily explained by matching the total surface area of droplets and the total cross-section area of interfacial stabilizers [25] : where ρ is the specific gravity of stabilizers with respect to the droplet phase, η is the porosity of interfacial packing and τ n is packing thickness. Conformation of experimental data to equation (1) indicates that fulfiling the interfacial area requirement for accommodating all stabilizer particles is an important determinant of droplet size. We further compare d n ( n >0) with d 0 , revealing a linear relationship between them: as shown in Fig. 2g–i . The scaling factor k n is estimated from the slope of linear regression. For n =1, 2 and 3, k 1 ≈1.6, k 2 ≈2.5 and k 3 ≈3.4 for all three emulsion systems. The conservation of k n 's among different emulsion systems suggests the presence of a univeral mechanism that controls the evolution of droplet size. Evolution of droplet size through multi-body coalescence To elucidate the mechanism of size evolution for Pickering droplets, we first focus on the mean diameter of deconvoluted droplet population without considering dispersion of the population. As shown in Fig. 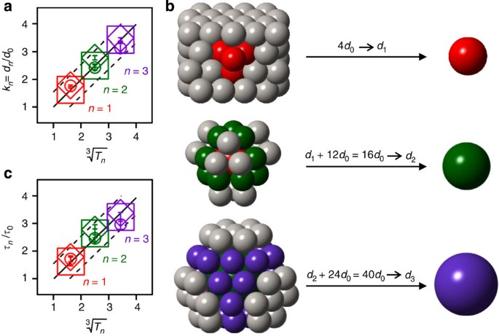Figure 3: Scaling of Pickering droplet diameters according to the tetrahedral number sequence. (a) Correlation of the scaling factorkn=dn/d0(n=1, 2, 3) with the cubic root of four times the tetrahedral number,Tn. (b) Formation ofdndroplets from the coalescence of onedn−1droplet (nodn−1droplet forn=1) and (Tn−Tn−1)d0droplets in face-centred close packing. Note: droplets coloured in grey do not participate in coalescence. (c) Increase of interfacial particle thickness after coalescence. Extra-large symbols inaandcare used for clarity of presentation: squares, latex particle-stabilized water droplets in dodecane; diamonds, silica particle-stabilized 1,2-dichlorobenzene droplets in water; circles, carbon nanotube-stabilized water droplets in dodecane. Solid lines inaandcare least-square regressions (R2=0.99). Dashed lines are 95% confidence intervals. Error bars represent s.e. 3a (see Supplementary Table 1 for data), k n equals the cubic root of four times the corresponding tetrahedral number, T n : Figure 3: Scaling of Pickering droplet diameters according to the tetrahedral number sequence. ( a ) Correlation of the scaling factor k n = d n / d 0 ( n =1, 2, 3) with the cubic root of four times the tetrahedral number, T n . ( b ) Formation of d n droplets from the coalescence of one d n −1 droplet (no d n −1 droplet for n =1) and ( T n − T n −1 ) d 0 droplets in face-centred close packing. Note: droplets coloured in grey do not participate in coalescence. ( c ) Increase of interfacial particle thickness after coalescence. Extra-large symbols in a and c are used for clarity of presentation: squares, latex particle-stabilized water droplets in dodecane; diamonds, silica particle-stabilized 1,2-dichlorobenzene droplets in water; circles, carbon nanotube-stabilized water droplets in dodecane. Solid lines in a and c are least-square regressions ( R 2 =0.99). Dashed lines are 95% confidence intervals. Error bars represent s.e. Full size image suggesting that a d n droplet has the same volume as T n d 0 droplets and thus is formed by their coalescence. For n =1, 2 and 3, T n =4, 16 and 40; therefore, the coalescence of these Pickering droplets is multi-body in nature. Multi-body coalescence requires droplets to be closely packed, which is facilitated by the density difference between water and oil in our experimental systems ( cf . Fig. 1g–i ) [26] . As illustrated in Fig. 3b and Table 1 , four nearest-neighbouring d 0 droplets form a tetrahedron in a face-centred close (FCC) packed ensemble. When all four droplets coalesce simultaneously, the new droplet has a diameter of , where T 1 =4. The d 1 droplet has 12 nearest d 0 neighbours in FCC, yielding a d 2 droplet after coalescing with the d 1 droplet: , where T 2 =4+12=16. Similarly, a d 3 droplet is formed by the coalescence of the d 2 droplet with its 24 nearest neighbours: , where T 3 =16+24=40. Table 1 Progression of coalescence in FCC packing*. Full size table We further examine multi-body coalescence by considering the material conservation of interfacial stabilizers before and after coalescence, which requires: By combining this equation with equation (2), we obtain: for constants ρ and η . Indeed, equation (5) holds for all three emulsion systems as illustrated in Fig. 3c (see Supplementary Table 2 for data). Polydispersity and size evolution In the analyses described above, we have assumed that each deconvoluted droplet population has a single diameter, d n ( n =0, 1, 2, 3), equal to the mean of the Gaussian fit of experimental data. For the 0th droplet population, this assumption can be validated by considering that d 0 droplets are formed under vigorous shaking—an independent and identical process with a finite variance [27] . However, will the coalescence of normally distributed d 0 droplets produce normally distributed d n ( n >0) droplets? Coalescence progresses through the conservation of volume: According to equation (6), we can prove that the probability density function of d n is the T n -fold convolution power of the probability density function of (see Supplementary Note 1 for derivation), which cannot be evaluated analytically. To obtain the distribution of the n th droplet population, we resort to the Monte Carlo method, which computes one million d n values from randomly selected d 0 's using equation (6). The histograms of simulated d n 's ( n >0) are shown in Fig. 4a , along with the normally distributed 0th population. The histograms can be well-approximated by normal distributions (similarity to normality >99.8%, as measured by Kolmogorov–Smirnov statistic) [28] , [29] , confirming that the normal distribution is conserved through coalescence. The means of simulated d n 's are compared with those estimated from experimental data in Fig. 4b . The two data sets exhibit an excellent linear correlation with a near-unity slope of 1.01(±0.01) ( R 2 =0.96), validating the use of Gaussian fits to estimate d n 's. 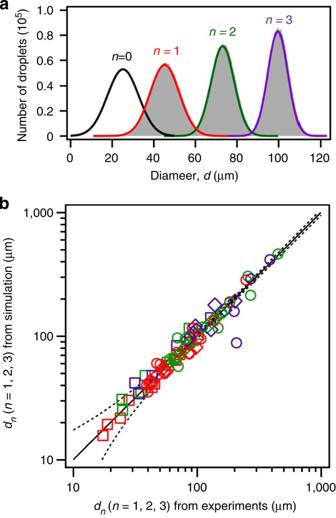Figure 4: Evolution of diameter distribution through coalescence examined by Monte Carlo simulation. (a) Evolution of the normal distribution ofd0with a mean of 25.3 μm and a s.d. of 7.5 μm (zeroth population inFig. 2a) through multi-body coalescence (grey shades, simulated populations; coloured curves, Gaussian fits). (b) Comparison of mean diameters ofdn's (n=1, 2, 3) obtained from fitting simulated data to Gaussian functions with those obtained from fitting experimental data to Gaussian functions. Symbols: squares, latex particle-stabilized water droplets in dodecane; diamonds, silica particle-stabilized 1,2-dichlorobenzene droplets in water; circles, carbon nanotube-stabilized water droplets in dodecane. Colours: red,n=1; green,n=2; purple,n=3. The solid line is obtained by linear regression (R2=0.96). Dashed curves bracket 95% confidence intervals. Figure 4: Evolution of diameter distribution through coalescence examined by Monte Carlo simulation. ( a ) Evolution of the normal distribution of d 0 with a mean of 25.3 μm and a s.d. of 7.5 μm (zeroth population in Fig. 2a ) through multi-body coalescence (grey shades, simulated populations; coloured curves, Gaussian fits). ( b ) Comparison of mean diameters of d n 's ( n =1, 2, 3) obtained from fitting simulated data to Gaussian functions with those obtained from fitting experimental data to Gaussian functions. Symbols: squares, latex particle-stabilized water droplets in dodecane; diamonds, silica particle-stabilized 1,2-dichlorobenzene droplets in water; circles, carbon nanotube-stabilized water droplets in dodecane. Colours: red, n =1; green, n =2; purple, n =3. The solid line is obtained by linear regression ( R 2 =0.96). Dashed curves bracket 95% confidence intervals. Full size image Coalescence probability and interparticle force Although Pickering droplets prepared with different stabilizers coalesce following the same tetrahedral sequence, the selection of stabilizer can, however, affect coalescence probability. This is revealed by examining the variation of relative abundance N n / N T ( n =0, 1, 2, 3) of each droplet population with α , as shown in Fig. 5 . Here N n is the number of d n droplets estimated by integrating the n th Gaussian fit and . As α increases, N n / N T ( n >0) increases at the expense of N 0 / N T for latex and silica-stabilized droplets ( Fig. 5a,b ), indicating that the addition of stabilizers promotes coalescence. For CNT-stabilized droplets ( Fig. 5c ), the opposite is observed, revealing improved stability of d 0 droplets and suppressed coalescence with the addition of CNTs. 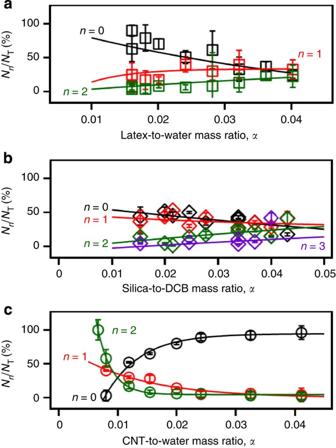Figure 5: Relative abundances of Pickering droplets from different normal populations. (a) Latex particle-stabilized water droplets in dodecane (b) Silica particle-stabilized 1,2-dichlorobenzene (DCB) droplets in water. (c) Carbon nanotube (CNT)-stabilized water droplets in dodecane.is the total number of droplets from all populations. Curves are regressions to exponential functions (R2>0.8). Error bars represent the standard deviation of the data. Figure 5: Relative abundances of Pickering droplets from different normal populations. ( a ) Latex particle-stabilized water droplets in dodecane ( b ) Silica particle-stabilized 1,2-dichlorobenzene (DCB) droplets in water. ( c ) Carbon nanotube (CNT)-stabilized water droplets in dodecane. is the total number of droplets from all populations. Curves are regressions to exponential functions ( R 2 >0.8). Error bars represent the standard deviation of the data. Full size image To understand why coalescence is promoted by latex and silica particles but suppressed by CNTs, we divide coalescence into two consecutive processes: packing and fusion, as illustrated in Fig. 6 . Packing presses d 0 droplets together and transforms them from spheres to rounded polyhedrons [30] . 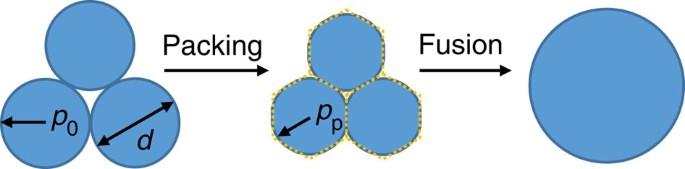Figure 6: Two consecutive processes of coalescence. Packing presses droplets together and transforms them from spheres to rounded polyhedrons. Fusion between droplets then occurs with the rupture of the separating liquid film to complete coalescence. To pack droplets sufficiently close for coalescence, Laplace pressure p 0 must be overcome by the external pressure provided by the droplets’ weight, P : Figure 6: Two consecutive processes of coalescence. Packing presses droplets together and transforms them from spheres to rounded polyhedrons. Fusion between droplets then occurs with the rupture of the separating liquid film to complete coalescence. Full size image where γ is interfacial tension. Fusion between droplets then happens with the rupture of the separating liquid film, which requires the internal pressure of polyhedral droplets, p p , to exceed the disjoining pressure of the film, Π (a property of the continuous phase) [31] , [32] : where C is a constant related to droplet packing fraction. The interfacial tension includes contributions from both stabilizer-wrapped droplets, γ d , and interactions between interfacial stabilizers, γ s : For stabilized droplets [2] , where γ ow is the oil–water interfacial tension and θ is the contact angle formed by the continuous phase, the stabilizer surface and the droplet phase. According to equation (10), γ d is constant for a given emulsion system; therefore, γ varies with γ s . γ s can arise from the electrostatic repulsion between interfacial stabilizers. Latex particles, silica particles and CNTs are all negatively charged, as confirmed by their negative zeta potentials in water (latex, −18(±7) mV; silica, −21(±7) mV; CNTs, −13(±1) mV). Charge-induced repulsion, γ cp , pushes stabilizer particles away from one another, reducing interfacial tension that pulls stabilizers together (that is, γ s =− γ cp <0): An indication of interparticle repulsion is the random close packing [33] patterns formed by latex and silica particles at the oil–water interface and revealed by confocal laser scanning microscopy, as shown in Fig. 7a–c and d–f , respectively. With low γ , equation (7) is readily fulfiled. The probability of coalescence is thus controlled by the difference between p p and Π according to equation (8). As α increases, d 0 decreases according to equation (1). This leads to an increase of p p , improving the chances of overcoming Π to coalesce and produce more d n ( n >0) droplets at greater α ( cf . Fig. 5a,b ). 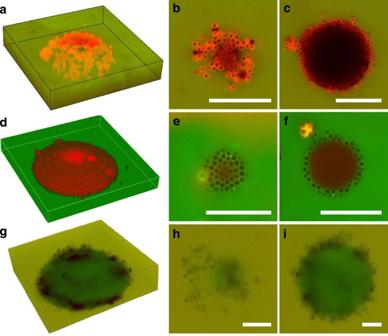Figure 7: False-colour confocal laser scanning micrographs of interfacial stabilizers. Images obtained with different stabilizers are organized in rows: (a–c) latex particle-stabilized water droplets in dodecane, (d–f) silica particle-stabilized 1,2-dichlorobenzene droplets in water and (g–i) carbon nanotube-stabilized water droplets in dodecane. Different types of images are organized in columns: (a,d,g) three-dimensional reconstructions of spherical caps, (b,e,h) cross-sections at the tops of spheres and (c,f,i) cross-sections below the tops. Note: the diameter of individual carbon nanotubes is much smaller than the imaging resolution (ca. 300 nm); therefore, individual nanotubes and bundles of a few nanotubes are not visually resolved. Mass ratio between droplets and the continuous phase: (a–c), 0.0667; (d–f), 0.0650 and (g–i), 0.0667. Stabilizer-to-droplet mass ratio: (a–c), 0.02; (d–f), 0.03 and (g–i), 0.01. Scale bars, 10 μm. Figure 7: False-colour confocal laser scanning micrographs of interfacial stabilizers. Images obtained with different stabilizers are organized in rows: ( a – c ) latex particle-stabilized water droplets in dodecane, ( d – f ) silica particle-stabilized 1,2-dichlorobenzene droplets in water and ( g – i ) carbon nanotube-stabilized water droplets in dodecane. Different types of images are organized in columns: ( a , d , g ) three-dimensional reconstructions of spherical caps, ( b , e , h ) cross-sections at the tops of spheres and ( c , f , i ) cross-sections below the tops. Note: the diameter of individual carbon nanotubes is much smaller than the imaging resolution (ca. 300 nm); therefore, individual nanotubes and bundles of a few nanotubes are not visually resolved. Mass ratio between droplets and the continuous phase: ( a – c ), 0.0667; ( d – f ), 0.0650 and ( g – i ), 0.0667. Stabilizer-to-droplet mass ratio: ( a – c ), 0.02; ( d – f ), 0.03 and ( g – i ), 0.01. Scale bars, 10 μm. Full size image Different from latex and silica particles, CNTs form an extended network at the oil–water interface, as revealed by the confocal micrographs shown in Fig. 7g–i . Formation of the network can be attributed to strong π–π attractions between individual nanotubes, which overtake electrostatic repulsions between them (that is, γ s = γ π–π − γ cp >0) [6] , [34] : With high γ , equation (8) is readily fulfiled, leaving the control of coalescence probability to equation (7). As α increases, d 0 decreases and p 0 increases, resulting in a decrease of coalescence and minimal amounts of d n ( n >0) droplets with large α ( cf . Fig. 5c ). We have shown that closely packed Pickering droplets can coalesce through a multi-body mechanism. We hypothesize that the determining factor of multi-body coalescence is the presence of stabilizers at the oil–water interface, which slows down coalescence. In ordinary emulsions where droplets are stabilized by surfactant molecules or ions, coalescence happens rapidly between two droplets [35] , [36] . Recent measurements have, however, shown that coalescence between two particle-stabilized droplets is orders of magnitude slower [37] . The extended transition time provides an opportunity for all of the nearest neighbours to be involved in a single coalescence event once coalescence is initiated between two droplets. We formulate the multi-body coalescence theory in the FCC configuration. If Pickering droplets are packed in the hexagonal close packing (HCP) configuration, the number of droplets involved in the first coalescence event is the same as in FCC but decreases gradually for the second and third events, as illustrated in Table 2 . The k n values for HCP are 1.6, 2.4 and 2.5 compared with 1.6, 2.5 and 3.4 for FCC. According to experimentally determined k n 's, the packing of Pickering droplets is better represented by FCC. Nonetheless, multi-body coalescence requires only short-range ordering because significant coalescence occurs in the first few coordination shells surrounding an interstitial void. In the longer range, the lack of organization, such as that in random close packing [33] , should not affect the outcome of multi-body coalescence in Pickering emulsions. Table 2 Progression of coalescence in HCP*. Full size table Reagents Reagent-grade chemicals were purchased from Sigma-Aldrich and Fisher Scientific except where otherwise stated. Deionized (DI) water (18.2 MΩ cm −1 ) used in solution making, washing and rinsing was generated using a Millipore system (Billerica, MA, USA) on site. We prepared Pickering emulsions by shaking and standing (see below) [20] . Latex particle-stabilized water droplets in dodecane Latex particles were obtained by drying an aqueous solution in vacuum overnight. The particles were then dispersed in dodecane (99%, TCI America) at various concentrations. To make Pickering emulsions, 50 μl DI water was added to 1 ml dodecane. The mixture was shaken by hand vigorously for 10 min and then left standing on bench for 10 min. Silica particle-stabilized DCB droplets in water Silica particles were first coated with (3-aminopropyl)trimethoxysilane (APTMS, 97%) to modify their surface wettability [38] . To do so, 0.1 ml particle solution (10 wt%) was dried in an oven at 120 °C overnight and was then mixed with 10 ml toluene (≥99.8%) and 100 μl APTMS. The mixture was shaken for 2 h. The particles were washed with toluene five times and with ethanol three times. The particles were then dried in an oven overnight to remove residual ethanol and immersed in water before use. To make a Pickering emulsion, 50 μl 1,2-DCB (99%, Alfa Aesar) was added to 1 ml DI water with different concentrations of silica particles. The mixture was shaken by hand vigorously and left standing undisturbed following the same procedure for making latex-stabilized emulsions. CNT-stabilized water droplets in dodecane Magnetite-decorated CNTs were prepared using multi-walled CNTs synthesized by chemical vapour deposition [6] . Catalysts were removed by washing with nitric acid. CNTs were then decorated with 10-nm magnetite nanoparticles using the polyol reduction method [39] . To make a CNT-stabilized Pickering emulsion, CNTs were dispersed in 10 ml water by sonication for 10 min, followed by an addition of 0.5 ml dodecane. The mixture was shaken and left standing quiescently following the same protocol for making latex and silica-stabilized emulsions. Optical microscopy Diameters of particle-stabilized droplets were measured using images taken by an optical microscope (Motic BA300POL). To do so, emulsions were poured on either glass (for silica-stabilized droplets) or plastic (for latex and CNT-stabilized droplets) Petri dishes. The emulsions were then diluted with the corresponding continuous phases to minimize droplet overlapping in the imaging field. For each sample, ~30 images were taken randomly with a × 10 objective lens (resolution: 1.25 μm per pixel). Diameters were measured using software ImageJ [40] . A few droplets stabilized by silica particles (<5%) were found at the arrested coalescence state with non-spherical shapes ( Supplementary Fig. 2 ). They were excluded in subsequent diameter analyses. Confocal laser scanning microscopy Interfacial stabilizers were visualized using a confocal laser scanning microscope (Nikon A1R) equipped with a × 100 Plan Apo total internal reflection fluorescence objective lens. The oil phases were illuminated using oil-soluble Nile red. Water was illuminated using Alex Fluor 488. Concentrations of the fluorescent dyes were: latex particle-stabilized water droplets in dodecane, 0.001 mM Alex Fluor 488 in water and 0.1 mM Nile red in dodecane; silica particle-stabilized DCB droplets in water, 0.03 mM Nile red in DCB and 0.01 mM Alex Fluor 488 in water; CNT-stabilized water droplets in dodecane, 0.01 mM Alex Fluor 488 in water and 0.03 mM Nile red in dodecane. The oil-in-water emulsion stabilized by silica particles was imaged using a custom-made hydrophilic glass reservoir. To image water-in-oil emulsions stabilized by latex particles and CNTs, the reservoir was treated with a 1:100 octadecyltrichlorosilane toluene solution to create a hydrophobic coating before use. Measurement of particle surface charge Zeta potentials of latex particles, silica particles and CNTs were measured using a ZetaPlus analyzer (Brookhaven Instruments) in water at concentrations of 0.2 mg l −1 , 0.2 mg l −1 and 0.12 mg l −1 , respectively. Water pH was adjusted according to the conditions in corresponding emulsions. Latex particles and CNTs were dispersed in water in equilibrium with atmospheric carbon dioxide at pH 5.6. Silica particles were dispersed in dilute sodium hydroxide solution at pH 7.0. Before measurements, stabilizer suspensions were sonicated for 30 min. For each stabilizer, five measurements were made. How to cite this article : Wu, T. et al . Multi-body coalescence in Pickering emulsions. Nat. Commun. 6:5929 doi: 10.1038/ncomms6929 (2015).